Planar hexagonal B36as a potential basis for extended single-atom layer boron sheets Boron is carbon’s neighbour in the periodic table and has similar valence orbitals. However, boron cannot form graphene-like structures with a honeycomb hexagonal framework because of its electron deficiency. Computational studies suggest that extended boron sheets with partially filled hexagonal holes are stable; however, there has been no experimental evidence for such atom-thin boron nanostructures. Here, we show experimentally and theoretically that B 36 is a highly stable quasiplanar boron cluster with a central hexagonal hole, providing the first experimental evidence that single-atom layer boron sheets with hexagonal vacancies are potentially viable. Photoelectron spectroscopy of B 36 − reveals a relatively simple spectrum, suggesting a symmetric cluster. Global minimum searches for B 36 − lead to a quasiplanar structure with a central hexagonal hole. Neutral B 36 is the smallest boron cluster to have sixfold symmetry and a perfect hexagonal vacancy, and it can be viewed as a potential basis for extended two-dimensional boron sheets. Soon after the discovery of carbon nanotubes [1] , analogous boron nanotubes were proposed [2] , [3] . However, a perfectly planar triangular lattice made of the boron nanotubes is unstable and instead adopts a rather buckled form [4] , [5] , [6] , [7] . Recent computational studies suggest that a triangular planar boron lattice with hexagonal vacancies is more stable [8] , [9] , which would be suitable to form the putative boron nanotubes and it underlies the stability of the proposed B 80 fullerene [10] . However, there has been no experimental evidence for the viability of this newly proposed planar boron sheet. Joint experimental and computational studies over the past decade have shown that boron clusters are planar or quasiplanar at large sizes [11] , [12] , [13] , [14] , [15] , [16] , [17] , [18] , [19] , [20] , [21] , in contrast to bulk boron where three-dimensional (3D) cages are prevalent. Boron clusters with a triangular lattice have invariably found to exhibit out-of-plane distortions [12] , [13] , [14] , [15] , [16] , [17] , [19] , [20] , [21] . Tetragonal or pentagonal defects are often found in truly planar boron clusters up to 23 atoms [12] , [17] , [18] , [19] , [20] . Here we report the discovery of a quasiplanar boron cluster with sixfold symmetry and a perfect central hexagonal hole, providing the first experimental evidence that large-scale planar boron sheets with hexagonal vacancies are potentially viable. This joint photoelectron spectroscopy (PES) and theoretical study shows that the B 36 – cluster is quasiplanar with a central hexagonal hole. Neutral B 36 is found to be a highly stable cluster with perfect C 6v hexagonal symmetry. Extension of this cluster would give rise to the planar boron sheets with hexagonal vacancies [8] , [9] , [22] , [23] . PES of the B 36 – cluster Boron cluster anions with up to 24 atoms have been investigated previously [11] , [12] , [13] , [16] , [17] , [18] , [19] , [20] , [21] . The PES spectra became more congested and complicated for clusters larger than 20 atoms [19] , [20] , [21] , presenting considerable challenges for both computational global minimum searches and comparison between experiment and theory. However, we found that the spectrum of B 36 – ( Fig. 1a ) is special, showing an unusually low electron-binding energy and well-resolved spectral features in the low binding energy side. We also measured the spectrum at 266 nm (not shown) with slightly higher resolution. The adiabatic detachment energy of 3.12 eV measured from the sharp onset of the first detachment band X in the 266 nm spectrum also represents the electron affinity (EA) of neutral B 36 . It is surprising that the EA of B 36 is even smaller than that of B 22 (3.34 eV) (ref. 20 ) or B 24 (3.55 eV) (ref. 21 ), since the EA generally increases with increasing cluster size. The low EA of B 36 is a result of the large energy gap, as revealed by the X–A separation, suggesting that neutral B 36 is a highly stable cluster with a large energy gap between its highest occupied (HOMO) and lowest unoccupied (LUMO) molecular orbitals. The weak feature X′ observed in Fig. 1a is due to contributions of a low-lying isomer ( vide infra ). 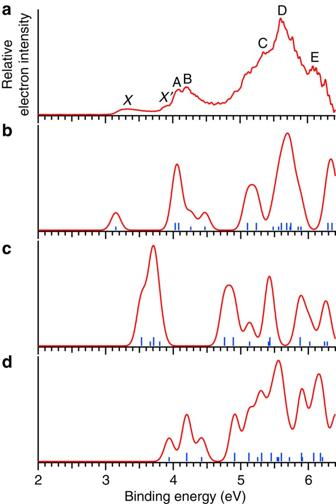Figure 1:Photoelectron spectroscopy of B36–and comparison with simulation. (a) The experimental spectrum at 193 nm. (b) The simulated spectrum for the global minimum quasiplanar structure with a hexagonal hole (I inFig. 2a). (c) The simulated spectrum for the tubular isomer (II inFig. 2a). (d) The simulated spectrum for the quasiplanar structure with two holes (III inFig. 2a). The vertical bars in the simulated spectra represent the calculated VDEs. The simulated spectra were obtained by fitting the VDEs with a unit area Gaussian function of 0.05 eV width. The vertical detachment energies (VDEs) of the observed detachment transitions are given in Supplementary Table 1 . Figure 1: Photoelectron spectroscopy of B 36 – and comparison with simulation. ( a ) The experimental spectrum at 193 nm. ( b ) The simulated spectrum for the global minimum quasiplanar structure with a hexagonal hole (I in Fig. 2a ). ( c ) The simulated spectrum for the tubular isomer (II in Fig. 2a ). ( d ) The simulated spectrum for the quasiplanar structure with two holes (III in Fig. 2a ). The vertical bars in the simulated spectra represent the calculated VDEs. The simulated spectra were obtained by fitting the VDEs with a unit area Gaussian function of 0.05 eV width. Full size image VDEs are usually measured from the peak maxima from PES spectra. For small clusters or simpler systems, PES bands are well separated and each band represents a single detachment transition. In the current case, bands X and A are well resolved and they should each correspond to a single electron detachment channel, as given in Supplementary Table 1 . The VDEs for bands X (3.3. eV) and A (4.08 eV) are directly obtained from the band maximum in each case. Band B is relatively broad, which is likely a result of several overlapping detachment transitions. Consequently, a range of energy (4.2–4.5 eV) is given for band B in Supplementary Table 1 . Following an energy gap, more congested detachment features are observed above 5 eV, suggesting a high density of electronic states. The label C is given to represent the signals from about 5.1–5.4 eV. An intense band D is observed at ~5.6 eV, which is also likely a result of overlapping detachment transitions. The sharp spikes on the higher binding energy side of band D cannot be assigned as individual detachment transitions because of the relatively low signal-to-noise ratios in this part of the spectrum. Finally, the label E represents the broad signals around 6.1 eV. Hence, all the labels from B to E do not represent individual detachment transitions and they are solely for the sake of discussion. The congested detachment transitions for such a large cluster are expected, as borne out from comparisons with the theoretical results ( infra vide ). The broad X band suggests a significant structural change from the anion to the neutral ground state. Despite the congested spectral features in the higher binding energy side, the relatively simple spectral pattern in the low binding energy side and the large HOMO–LUMO gap indicate that neutral B 36 should be a highly symmetric cluster. Computational results We searched for energetically low-lying isomers of B 36 – with the Cartesian Walking (CW) method [19] and TGmin [24] , a constrained Basin–Hopping code using energies from density functional theory (DFT). Among the 3,000 or so trial structures in our search, a quasiplanar pseudo-C 6v structure with a hexagonal hole was found to be much more stable than any other isomers. We also considered a ring-type structure, which was shown to be stable for large boron clusters [13] , [15] , [20] , [25] , [26] , [27] . Refined geometry optimizations and vibrational frequency calculations were performed using DFT method with the hybrid PBE0 [28] exchange-correlation functional with the 6-311G* basis set [29] on all structures within 70 kcal mol −1 of the pseudo-C 6v global minimum structure ( Supplementary Fig. 1 ). Zero-point energy corrections were included for all the isomers at the PBE0/6-311G* level. The effect of including the zero-point corrections was small for isomers of similar structures but could be substantial (shifting relative energy values by around 2 kcal mol −1 ) for isomers of different structural types (that is, 2D versus 3D). We found that the hexagonal global minimum structure of B 36 – and its corresponding neutral species exhibit C 2v (pseudo-C 6v ) and C 6v symmetries, respectively ( Fig. 2 ). The nearest isomers of B 36 – , a triple ring and a double-hole quasiplanar structure, lie 10.5 and 14.7 kcal mol −1 higher in energy at the PBE0 level of theory. Our global search also led to a number of other 3D structures, such as cage-like structures and two-layer structures, which are all much higher in energy (see Supplementary Fig. 1 ). Cartesian coordinates of the three lowest-lying structures of B 36 – and B 36 ( Fig. 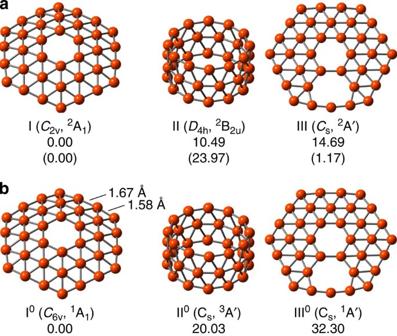Figure 2:The global minimum and low-lying isomers of B36−and B36. (a) Relative energies for the isomers of B36−are given in kcal mol−1at the PBE0/6-311G* and CCSD/6-31+G*//PBE0/6-311G* (in parenthesis) levels of theory. (b) Relative energies for the isomers of B36are given in kcal mol−1at the PBE0/6-311G* level of theory. All energies have been corrected for zero-point energies at the PBE0/6-311G* level. 2 ) are given in Supplementary Table 2 . Figure 2: The global minimum and low-lying isomers of B 36 − and B 36 . ( a ) Relative energies for the isomers of B 36 − are given in kcal mol −1 at the PBE0/6-311G* and CCSD/6-31+G*//PBE0/6-311G* (in parenthesis) levels of theory. ( b ) Relative energies for the isomers of B 36 are given in kcal mol −1 at the PBE0/6-311G* level of theory. All energies have been corrected for zero-point energies at the PBE0/6-311G* level. Full size image Comparison of experimental and simulated spectra of B 36 – To confirm the global minimum of B 36 – , we compare its simulated spectrum with the experimental data in Fig. 1 and Supplementary Table 1 . The relatively simple spectral pattern can act as an electronic fingerprint. The overall simulated spectral pattern of the C 2v global minimum of B 36 – ( Fig. 1b ) is in good accord with the experimental spectrum. In particular, the calculated first and second VDEs are in excellent agreement with the experimental observation, confirming the large HOMO–LUMO gap observed and the unusually low EA of B 36 . The LUMO of the hexagonal B 36 (C 6v ) is doubly degenerate with e 2 symmetry ( Supplementary Fig. 2 ). The C 2v symmetry of B 36 – is, hence, due to the Jahn–Teller effect as a result of the occupation of the degenerate LUMO in the anion. The broad X band is consistent with a significant geometry change between the anionic and neutral B 36 , primarily involving the distortion of the hexagonal hole in the anion ( Supplementary Fig. 3 ). However, the higher binding energy side of the experimental spectrum ( Fig. 1a ) is complicated and is not reproduced well by the simulated spectrum of the C 2v global minimum of B 36 – ( Fig. 2b ). Furthermore, the weak peak labelled as X′ observed experimentally was not reproduced by the simulated spectrum of the C 2v B 36 – , consistent with the suggestion that it might be due to a low-lying isomer. We further tested the possibility of isomer contributions by computing the VDEs for the two lowest-lying isomers (II and III in Fig. 2a ), as presented in Fig. 1c,d and Supplementary Tables 3 and 4 , respectively. The first five detachment channels of the tubular isomer II are close to each other around 3.7 eV ( Fig. 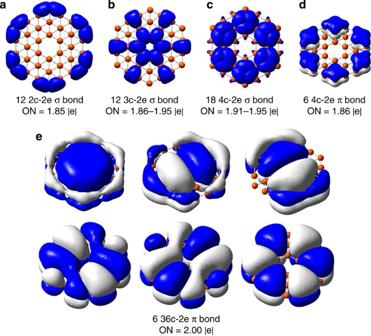Figure 3:Chemical bonding analysis for the hexagonal C6vstructure of B36. The analysis was performed using the AdNDP method33. ON stands for occupation number and is equal to 2.00 |e| (meaning a density of exactly two electrons) in the ideal case. 1c and Supplementary Table 3 ), corresponding to the gap region between bands X and A. Thus, isomer II can be ruled out as a discernible contributor to the observed spectrum. On the other hand, the first detachment channel of isomer III is in good agreement with the X′ band ( Fig. 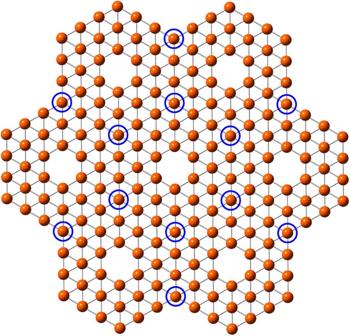Figure 4:Relationship between B36and borophene. A schematic view of part of an extended one-atom-thick boron sheet, named borophene, as constructed from the planar hexagonal B36unit. The circles represent the apex atoms in the B36unit that are shared by three units. Removal of these atoms would lead to the α-sheet8. 1d and Supplementary Table 4 ). Furthermore, the second and third detachment channels of isomer III agree well with the broad band B, and the higher detachment channels of isomer III also seem to coincide with the congested higher binding energy part of the experimental spectrum. However, isomer III is 14.7 kcal mol −1 higher than the global minimum isomer I at the PBE0 level and it is not expected to be populated in any significant amount because our cluster beam is expected to be fairly cold. Under similar experimental conditions, van der Waals complexes of Ar and anionic gold clusters were observed, [30] indicating a vibrational temperature of <200 K. We then calculated the energies of the first three isomers using the more accurate, but computationally more demanding, CCSD level [31] of theory with the 6-31+G* basis set [32] ( Fig. 2a ) and found that the double hole quasiplanar isomer III became more stable, only 1.17 kcal mol −1 above the global minimum C 2v isomer. Thus, isomer III would be expected to be substantially populated experimentally. The tubular isomer became 23.97 kcal mol −1 above the global minimum and its presence in our experiment can be safely ruled out. The combination of the simulated spectra of isomers I and III and their close energetic stability provide a much satisfying agreement with the experimental observations, lending considerable credence for the identified C 2v global minimum with a hexagonal hole for B 36 – . The electronic structure and stability of the hexagonal B 36 Our calculations show that neutral B 36 has perfect hexagonal symmetry (C 6v ) and is overwhelmingly stable relative to the closest-lying isomers II or III ( Fig. 2b ). The hexagonal B 36 has an out-of-plane distortion with the shape of a bowl, and its valence molecular orbitals are shown to be similar to those of a planar structure optimized with D 6h constraint. DFT calculations at the PBE0/6-311G* level of theory show that the D 6h structure is a saddle point at ~9 kcal mol −1 above the C 6v global minimum. The peripheral B–B bonding is enhanced upon shortening the B–B distance, which induces the out-of-plane bending in B 36 to the C 6v bowl shape. The bowl height is 1.16 Å with two different types of peripheral B–B distances, which are reduced from 1.61 and 1.72 Å in D 6 h to 1.58 and 1.67 Å, respectively, in the C 6v structure (I 0 in Fig. 2b ). The shorter bond length occurs between the six apex B atoms and their neighbours (1.58 Å), while the remaining six peripheral B–B bonds are slightly longer (1.67 Å). We analysed the chemical bonding of the hexagonal C 6v B 36 as well as the D 6h form of the cluster using adaptive natural density partitioning (AdNDP) [33] , which localizes the computed density matrix into n -centre two-electron ( n c-2e) bonds, with n ranging from one to the total number of atoms in the molecule. The AdNDP analysis of the D 6h structure is shown in Fig. 3 ; an analysis of the C 6v structure leads to similar results. AdNDP reveals 12 2c-2e σ bonds describing the shorter B–B bonds involving the six apex B atoms, 12 3c-2e σ bonds, 18 4c-2e σ bonds, six 4c-2e π bonds and six completely delocalized 36c-2e π bonds. The bonding pattern suggests that the B 36 cluster can be viewed as six hexagonal B 7 (B©B 6 ) units bound together by the 12 3c-2e σ bonds and the six 36c-2e π bonds. The totally delocalized 36c-2e π bonds in B 36 are interesting, which may be partly responsible for the remarkable stability of this hexagonal boron cluster. Figure 3: Chemical bonding analysis for the hexagonal C 6v structure of B 36 . The analysis was performed using the AdNDP method [33] . ON stands for occupation number and is equal to 2.00 |e| (meaning a density of exactly two electrons) in the ideal case. Full size image The necessity of hexagonal holes in stable planar 2D boron sheets was analysed in detail by Tang and Ismail-Beigi [8] , who considered the electronic structures of a graphene-like hexagonal boron sheet and a triangular boron lattice. They also showed a model B 32 cluster with a hexagonal hole to be more stable than a double ring structure. To explore the effect of the hexagonal hole on the stability of the B 36 cluster, we also optimized the structure of a B 37 cluster with C 6v symmetry by filling the hexagonal hole in B 36 with an extra B atom. We found that this B 37 cluster with a triangular lattice has an open-shell quartet electronic state with a (a 1 ) (ref. 1 ) (e 2 ) (ref. 2 ) configuration. The optimized structure is found to have changed significantly from the C 6v B 36 cluster: buckling of certain boron atoms was observed in contrast to the smooth bowl shape in the parent B 36 . This buckling of the B 37 cluster is similar to the buckled 2D boron sheets with triangular lattices [4] , [5] , [6] , [7] , [8] . The calculated atomization energy per B atom at the PBE/TZ2P level [34] , [35] reduces from 130.8 kcal mol −1 (5.67 eV per atom) for the C 6v B 36 cluster to 128.9 kcal mol −1 (5.59 eV per atom) for the C 6v B 37 cluster. Interestingly, the difference in the atomization energy (~0.08 eV per atom) between the hexagonal C 6v B 36 and the buckled B 37 cluster is also similar to that of the most stable 2D boron sheet with hexagonal holes and the buckled triangular 2D sheet (~0.11 eV per atom) at the DFT GGA level [8] . The relationship of the hexagonal B 36 and 2D boron sheets The hexagonal hole in the B 36 cluster is reminiscent of the hexagonal vacancies in the 2D boron sheets recently predicted [8] , [9] . The B 36 cluster can be viewed as the analogous boron unit of the hexagonal C 6 unit in graphene to form extended graphene-like boron nanostructures with hexagonal holes, as shown schematically in Fig. 4 . The structure shown in Fig. 4 represents a hexagonal hole density of η =1/27 (one vacancy per 27 lattice sites in a triangular lattice), as defined for the 2D boron sheet [8] . The structure in Fig. 4 is constructed by sharing a row of B atoms between two neighbouring B 36 units. The apex atoms (circled in Fig. 4 ) are shared by three neighbouring B 36 units. If these atoms are removed, one arrives at the more stable α-sheet with η =1/9 (refs 8 , 9 ). Interestingly, a B 30 model has been used to analyse the bonding in the proposed α-sheet [36] , which is equivalent to removing all six apex B atoms in the B 36 cluster. Hence, the B 36 cluster can be viewed as the embryo for the various proposed stable 2D boron sheets. Figure 4: Relationship between B 36 and borophene. A schematic view of part of an extended one-atom-thick boron sheet, named borophene, as constructed from the planar hexagonal B 36 unit. The circles represent the apex atoms in the B 36 unit that are shared by three units. Removal of these atoms would lead to the α-sheet [8] . Full size image However, it should be pointed out that Fig. 4 is only schematically showing the relationship between the hexagonal B 36 cluster and the stable 2D boron sheet. It does not represent the growth mechanism of the putative boron sheet, as it has been shown computationally that large boron clusters exhibit polymorphism with close-lying 3D cage-like structures [37] , [38] . Liu et al. [39] have considered computationally possible synthesis of 2D boron sheets on coinage metal surfaces as substrates, analogous to the synthesis of graphene. Thus, B 36 or other small boron clusters with hexagonal holes may serve as the nuclei for the formation of large-scale 2D boron sheets on the substrate. The present study provides the first experimental evidence for the viability of novel boron nanostructures with hexagonal vacancies. These structures can indeed exist and may be synthesized using appropriate substrates [39] . The potential large-scale synthesis of the new atom-thick boron nanosheets calls for an appropriate name: ‘borophene’ is proposed here, in analogy to graphene. The electronic structure of the 2D boron sheets can be either metallic or semiconducting, according to theoretical calculations [8] , [9] , [22] , [23] . Owing to the hexagonal holes, various chemical modifications are possible to tune the electronic and chemical properties of borophenes [40] , [41] . Thus, borophene may constitute a new class of atom-thick nanostructures complementary to graphene. Photoelectron spectroscopy The experiment was performed using a PES apparatus equipped with a magnetic-bottle photoelectron analyser and a supersonic cluster source [42] . Boron cluster anions (B x – ) were produced by laser vaporization of a hot-pressed boron target made of 10 B-enriched powder with a helium carrier gas seeded with 5% argon, which was shown previously to produce cold clusters [30] . The clusters were entrained in the carrier gas and underwent a supersonic expansion. Negatively charged clusters were extracted from the cluster beam and analysed by a time-of-flight mass spectrometer. Clusters of interest were mass-selected, decelerated and photodetached by a laser beam at 266 and 193 nm. The photoelectron spectra were measured using a magnetic-bottle PES analyser and calibrated by the known spectra of Au – and Bi – . The resolution (ΔEk/Ek) of the magnetic-bottle analyser was 2.5%—that is, 25 meV for 1 eV electrons. Computational and theoretical methods DFT global minimum searches were carried out using two methods, the CW method and a constrained Basin–Hopping method in the TGMin code [24] . The CW method has been described in detail elsewhere [19] . The CW search of B 36 – used DFT for energy evaluation, employing the PBE functional and the 3-21G basis set [43] from the Gaussian 09 program [44] . Within roughly 500 trial structures, a quasiplanar structure of near C 6v symmetry with a central hexagonal hole was found to be low in energy. We re-optimized all trial structures under 20 kcal mol −1 at the PBE0/3-21G level; the pseudo-C 6v structure remained the lowest in energy. Using the TGMin code we performed a more thorough search for the global minimum of B 36 – . The calculations were carried out using the DFT formalism with the PBE exchange-correlation functional and the Goedecker–Teter–Hutter pseudopotential [45] with the associated double-ζ valence plus polarization basis set [35] for boron via the CP2K program [46] . Among more than 2,500 possible structures produced by TGMin and the manually built tubular structures, we located a bowl-shaped pseudo-C 6v isomer with a hexagonal hole in the centre as the global minimum of B 36 – ( Fig. 1a ), in agreement with the CW result. Further analyses and geometry optimizations indicate that the actual symmetries of this anion and its neutral cluster are C 2v and C 6v , respectively. We further refined the energies by reoptimizing the geometries of low-lying isomers within 70 kcal mol −1 of the global minimum using DFT method with the hybrid PBE0 functional and the 6-311G* basis set from the Gaussian 09 program. Vibrational frequencies were calculated for each isomer and all the structures were ensured to be minima on the potential energy surface without imaginary frequencies. The re-optimized geometric structures and the PBE0 energies of the low-lying structures within 63 kcal mol −1 of the global minimum are given in Supplementary Fig. 1 . For more accurate relative energy assessment, single point calculations for the three lowest lying isomers were carried out using the CCSD formalism with the 6-31+G* basis set at their corresponding PBE0/6-311G* geometries using the Molpro software package [47] , [48] , [49] . We calculated the VDEs for the three low-lying structures to compare with the experimental photoelectron spectrum. The VDEs were computed using an approach named ΔSCF-TDDFT previously [50] , [51] . In this approach, the ground-state energies of the anions and the neutrals were calculated at the optimized geometries of the anions from the ΔSCF energy differences at the PBE0/6-311+G* level of theory, whereas the vertical excited-state energies of the electron-detached neutral species were obtained from TDDFT calculations at the geometries of the anions. These excitation energies were then added to the first VDE to approximate the high-lying VDEs. Only those neutral excited states with one-electron detachment from the anion ground state were chosen. The relative intensities used for the VDEs were assigned empirically on the basis of the spin multiplicities of the final states, one for singlet and two for triplet final states. The simulated PES spectra were constructed by fitting the distribution of the VDEs with unit-area Gaussian functions of 0.07 eV full width at half-maximum. This approach has been used extensively in elucidating the structures of size-selected clusters previously [16] , [17] , [18] , [19] , [20] , [21] . How to cite this article: Piazza, Z. A. et al. Planar hexagonal B 36 as a potential basis for extended single-atom layer boron sheets . Nat. Commun. 5:3113 doi: 10.1038/ncomms4113 (2014).